Common and rare variants associating with serum levels of creatine kinase and lactate dehydrogenase Creatine kinase (CK) and lactate dehydrogenase (LDH) are widely used markers of tissue damage. To search for sequence variants influencing serum levels of CK and LDH, 28.3 million sequence variants identified through whole-genome sequencing of 2,636 Icelanders were imputed into 63,159 and 98,585 people with CK and LDH measurements, respectively. Here we describe 13 variants associating with serum CK and 16 with LDH levels, including four that associate with both. Among those, 15 are non-synonymous variants and 12 have a minor allele frequency below 5%. We report sequence variants in genes encoding the enzymes being measured ( CKM and LDHA ), as well as in genes linked to muscular ( ANO5 ) and immune/inflammatory function ( CD163/CD163L1, CSF1, CFH, HLA-DQB1, LILRB5, NINJ1 and STAB1 ). A number of the genes are linked to the mononuclear/phagocyte system and clearance of enzymes from the serum. This highlights the variety in the sources of normal diversity in serum levels of enzymes. The release of intracellular enzymes into the serum is an indicator of tissue damage and physiological cell turnover. Thus, measurements of intracellular enzymes in serum are widely used to diagnose tissue damage, monitor its course and severity and gauge the effect of therapy. Creatine kinase (CK) is an enzyme, catalyzing the ATP-dependent phosphorylation of creatine that is important for energy buffering in tissues with variable energy demands, most notably skeletal and cardiac muscle [1] . Elevated serum CK levels can indicate tissue damage, and are observed in a number of pathological conditions, including statin-induced myopathy [2] . Monitoring changes in serum CK levels is therefore important in statin-treated patients who display muscle pain or weakness [3] , and in patients deemed at risk of rhabdomyolysis for various reasons [4] . Lactate dehydrogenase (LDH) is an enzyme with a ubiquitous expression [5] . It is responsible for catalyzing the anaerobic, nicotinamide adenine dinucleotide phosphate-dependent conversion of pyruvate to lactate, which is important during times of high muscular activity [6] . Serum CK and LDH levels were previously used as biomarkers to diagnose myocardial infarction. Because of low specificity, however, they have been replaced by troponin T and troponin I [7] , measured through high-sensitivity assays [8] . The heritability of LDH levels has been estimated between 40 and 50% (refs 9 , 10 ) and upwards of 38% for CK (ref. 11 ). Our own data indicates a 19.33 and 19.36% heritability for CK and LDH, respectively. A recently published genome-wide association study (GWAS) of 3,232,779 imputed variants in 3,412 statin users found two missense variants affecting serum CK levels, one in CKM (rs11559024) and one in LILRB5 (rs12975366) (ref. 12 ). An association of a variant in CD163 (rs7136716) with serum CK levels has also been reported [13] . To date, no systematic GWAS has been carried out to search for sequence variants influencing serum LDH levels. To search for common and rare variants that associate with CK or LDH levels, we tested variants detected in a large sequencing study in Iceland for association with these traits [14] . This unbiased approach has the potential to uncover previously unexpected molecular mechanisms regulating levels of this enzyme in serum. A thorough understanding of sequence variants influencing these biomarkers is important to improve the usefulness of their measurements, and in the assessment of tissue damage [15] . Summary of findings To search for sequence variants associating with mean serum levels of CK and/or LDH, we analysed 28.3 million variants, initially identified through whole-genome sequencing of 2,636 Icelanders and subsequently imputed into chip-typed individuals through long-range haplotype phasing [16] . Genotype probabilities were calculated for first and second-degree relatives of chip-typed individuals [17] . We tested for association between sequence variants and serum CK in 63,159 individuals (35,623 chip-typed and 27,536 with chip-typed first or second-degree relatives), and serum LDH in 98,585 individuals (52,581 chip-typed and 46,004 with chip-typed first- or second-degree relatives). We used methodology outlined by Sveinbjornsson et al . [18] to determine weighted genome-wide significance thresholds for different variant classes based on the total number of variants tested per class: loss-of-function ( N =6,476; P =2.6 × 10 −6 ); missense ( N =100,502; P =1.7 × 10 −7 ); and other ( N =23,854,999; P =7.0 × 10 −10 ). We found a total of 13 variants associated with CK, and 16 associated with LDH. 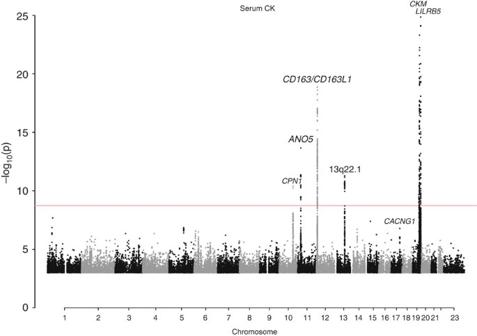Figure 1: Manhattan plot showing the seven loci harbouring genome-wide significant signals influencing serum CK levels in the Icelandic population. Variants are plotted by chromosomal position (xaxis) and −log10Pvalues (yaxis).Pvalues above 1 × 10−25are represented. Two loci (CKMandLILRB5) harbour variants withPvalues below this cutoff (rs11559024:P=1.8 × 10−115; rs12975366:P=6.5 × 10−44and rs393600:P=1.4 × 10−33). The red line indicates the threshold for genome-wide significance, determined by the number of tests performed (P=0.05/28.3 million=1.8 × 10−9). Of those, four were associated with both enzymes ( Table 1 , Figs 1 and 2 ). In total, all of the reported sequence variants explain 1.9% of CK variance, and 1.8% of LDH variance. Our results include replication of variants in CKM, LILRB5 and CD163 reported in GWASs of serum CK levels [12] , [13] . None of the variants showed more significant associations when alternate inheritance models were tested ( Supplementary Tables 2 and 3 ), and no additional variants were detected using these models. Table 1 Summary of single marker associations for CK ( N =63,159) and LDH ( N =98,585) in Iceland. Full size table Figure 1: Manhattan plot showing the seven loci harbouring genome-wide significant signals influencing serum CK levels in the Icelandic population. Variants are plotted by chromosomal position ( x axis) and −log 10 P values ( y axis). P values above 1 × 10 −25 are represented. Two loci ( CKM and LILRB5 ) harbour variants with P values below this cutoff (rs11559024: P =1.8 × 10 −115 ; rs12975366: P =6.5 × 10 −44 and rs393600: P =1.4 × 10 −33 ). The red line indicates the threshold for genome-wide significance, determined by the number of tests performed ( P =0.05/28.3 million=1.8 × 10 −9 ). 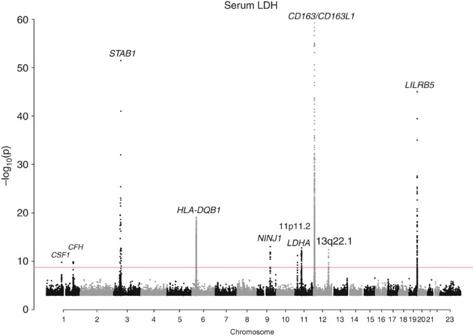Figure 2: Manhattan plot showing the 10 loci harbouring genome-wide significant signals influencing serum LDH levels in the Icelandic population. Variants are plotted by chromosomal position (xaxis) and −log10Pvalues (yaxis).Pvalues above 1 × 10−60are represented. One locus (CD163L1) harbours a variant withPvalue below this cutoff (rs4072797:P=9.9 × 10−89). The red line indicates the threshold for genome-wide significance, determined by the number of tests performed (P=0.05/28.3 million=1.8 × 10−9). Full size image Figure 2: Manhattan plot showing the 10 loci harbouring genome-wide significant signals influencing serum LDH levels in the Icelandic population. Variants are plotted by chromosomal position ( x axis) and −log 10 P values ( y axis). P values above 1 × 10 −60 are represented. One locus ( CD163L1 ) harbours a variant with P value below this cutoff (rs4072797: P =9.9 × 10 −89 ). The red line indicates the threshold for genome-wide significance, determined by the number of tests performed ( P =0.05/28.3 million=1.8 × 10 −9 ). Full size image Eleven of the variants are common (minor allele frequency (MAF)>5%), eight are of low frequency (MAF=0.5-5%) and five are rare (MAF<0.5%). Five loci contain several independent signals, associating with either one or both of the enzymes measured ( Fig. 3 ). For loci with multiple signals, we present P values and effects before and after adjusting for other significant markers at that locus ( Table 1 ). All variants correlated ( r 2 >0.6) with the variants we report are shown in the Supplementary Data 1 and Supplementary Figs 5–33 . 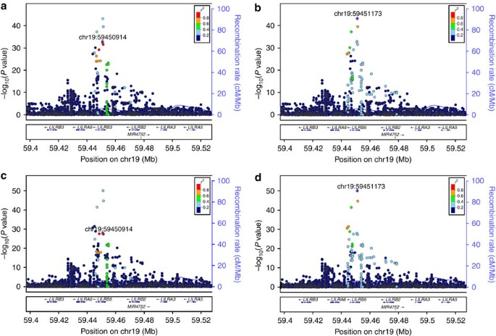Figure 3: Locus plots depicting variants at the LILRB5 locus associating with serum enzyme levels. Leading variants are labelled and shown in purple, other variants are coloured according to correlation (r2) with the leading marker (legend at top-right). −log10Pvalues are shown along the leftyaxis and correspond to the variants depicted in the plot. The rightyaxis shows calculated recombination rates at the chromosomal location, plotted as a solid blue line. (a) Association between the signal represented by rs393600 and serum CK levels. (b) Association between the signal represented by rs12975366 and serum CK levels. (c) Association between the signal represented by rs393600 and serum LDH levels. (d) Association between the signal represented by rs12975366 and serum LDH levels. Figure 3: Locus plots depicting variants at the LILRB5 locus associating with serum enzyme levels. Leading variants are labelled and shown in purple, other variants are coloured according to correlation ( r 2 ) with the leading marker (legend at top-right). −log 10 P values are shown along the left y axis and correspond to the variants depicted in the plot. The right y axis shows calculated recombination rates at the chromosomal location, plotted as a solid blue line. ( a ) Association between the signal represented by rs393600 and serum CK levels. ( b ) Association between the signal represented by rs12975366 and serum CK levels. ( c ) Association between the signal represented by rs393600 and serum LDH levels. ( d ) Association between the signal represented by rs12975366 and serum LDH levels. Full size image Most of the suspected genes are implicated in immune/inflammatory response, enzyme clearance or muscular function, but two encode subunits of the enzymes measured ( cis signals) and one encodes a protein that affects rates of CK clearance from plasma. Cis signals We observed variants in CKM and LDHA , genes that encode subunits of CK and LDH, respectively, with minor alleles that associate with a lower level of their corresponding serum enzyme levels. Enzymatic levels were measured by assessing quantity through enzymatic activity. Our results, therefore, indicate that these sequence variants act to either decrease the amount of the enzyme produced, or their catalytic ability. CKM Through a stepwise conditional analysis at 19q13.3, we found that four independent missense variants in CKM associate with serum CK levels. With one of these, rs11559024 [C] (MAF=2.15%, Glu83Gly), we replicated a reported association [12] . The associations of the remaining three low-frequency and rare missense variants are novel. Minor alleles of all four CKM variants have a large lowering effect on CK levels. We never observed more than one of the minor alleles on the same chromosome (all r 2 ≤2.2 × 10 −4 ; Supplementary Table 4 ). CKM encodes CK-M, one of two subunits of the CK dimer. Three isoforms of the enzyme exist, consisting of different combinations of CK-M and/or CK-B. Each isozyme has a unique expression profile; CK-MM is expressed in skeletal muscle, CK-MB in cardiac muscle and CK-BB in smooth muscle and the brain [19] . CK-MM typically accounts for the majority of serum CK (ref. 20 ). LDHA The missense variant rs116841148 [T] (MAF=0.652%, Ala147Ser) at 11p15.1 in LDHA associates with serum LDH levels ( Table 1 ). LDHA encodes the M subunit of the LDH enzyme, expressed in all but one of the five isozymes of LDH (ref. 21 ). CPN1 At 10q24.2, the low-frequency missense variant rs61751507 [T] (MAF=4.06%, Gly178Asp) in CPN1 associates with lower CK levels ( Table 1 ). CPN1 encodes carboxypeptidase N. This protein is expressed in blood, hydrolyzes CK-MM 1 ′s C-terminal lysine and converts CK-MM 1 , the enzyme‘s unaltered form as expressed in tissue, into either CK-MM 2 or CK-MM 3 . This hydrolyzation alters CK-MM’s isoelectric point and half-life without affecting properties such as enzymatic activity [22] , [23] . It is, therefore, plausible that if the variant in CPN1 induces a change in activity of carboxypeptidase N, it would affect CK-MM clearance rather than having a direct effect on enzymatic activity. Immune system genes associating with CK and/or LDH levels Seven loci harbouring variants associating with serum CK and/or LDH levels have genes that are likely to be responsible for the associations that are involved in immune or inflammatory response; CSF1 , CD163/CD163L1 , STAB1 , CFH , LILRB5 , HLA-DQB1 and NINJ1 . Three of these genes ( CSF1, CD163 and STAB1 ) have direct links to the clearance of products of cell lysis from the serum through the mononuclear phagocytic system (MPS) (refs 24 , 25 , 26 ). The remaining four implicated genes do not have a known link to enzyme clearance, although most are preferentially expressed in cells of the myeloid lineage. CSF1 At 1p13.3, the intronic variant rs333947 [A] (MAF=14.92%) in CSF1 associates with lower LDH levels ( Table 1 ). We observed no correlated coding variants ( r 2 >0.6) that could explain the association ( Supplementary Data 1 ). The position shows a high degree of evolutionary conservation (GERP (ref. 27 ) =4.83; Supplementary Table 5 ). CSF1 encodes human macrophage-specific colony stimulating factor, a cytokine necessary for the differentiation of monocyte lineage cells, including hepatic Kupffer cells (KCs) (ref. 24 ). In animal models, reducing KC numbers affects serum enzyme levels, including CK, LDH and aspartate transaminase (AST), without evidence of skeletal or liver damage [24] . Rs333947 [A] also associates with lower AST levels ( Supplementary Table 6 ). We also observed a suggestive association with CK levels. The associations we observed are consistent with CSF1 function and may indicate an increased macrophage activity, promoting faster clearance of serum enzymes. We assessed all sequence variants discussed in this paper for associations with AST levels ( Supplementary Table 6 ). Seven variants, including rs333947, associate with AST based on the number of tests performed ( P <0.05/25=2.0 × 10 −3 ). The direction of effect was always consistent; each allele either had an increasing or decreasing effect on the levels of all enzymes it associates with. CD163/CD163L1 At 12p13.31, the region containing CD163 and its paralog CD163L1 , we observed associations with CK and LDH levels ( Table 1 ). Two variants associated with both CK and LDH levels and four only with LDH levels. Two common variants associate with higher serum levels of CK and LDH; the intergenic variant rs7305678 [T] (MAF=16.16), and the intronic rs117692263 [C] (MAF=9.31%). Three low-frequency missense variants in the region associate solely with serum LDH levels; rs4072797 [T] (MAF=4.21%, Asp588Asn) and rs145411783 [A] (MAF=0.66%) in CD163L1 , and rs4883263 [T] (MAF=3.73%, Ile342Val) in CD163 . Finally, a common intergenic indel (chr12:7282745:0:TA MAF=21.13%) associates with LDH levels. CD163 encodes a scavenger receptor expressed on macrophages and monocytes, including KCs, that is responsible for uptake of the haemoglobin–haptoglobin complex from the bloodstream [25] . The CD163L1 gene, encoding the M160 receptor, is closely related to CD163 . The paralog is expressed by many of the same cells and has a sequence that is highly similar to that of CD163 (ref. 28 ), but does not have affinity for the same ligands as CD163 (ref. 25 ). Association of the intergenic variant rs7305678 with serum CK levels replicates a previously published association between a single marker, rs7136716 at the CD163 locus and serum CK levels in the Japanese [13] . Rs7136716 correlates with rs7305678 in both the Chinese/Japanese ( r 2 =0.85 [29] ) and Icelandic ( r 2 =0.75) populations, but is independent of other signals we report in the region. STAB1 At 3p21.1, the very rare missense variant rs150956780 [C] (MAF=0.078%, Val1522Leu) at a highly conserved site within STAB1 (GERP (ref. 27 )=4.56) associates with drastically lower serum LDH levels (effect=−1.526SD) ( Table 1 ). An association signal was observed across a large region and rs150956780 is more frequent outside of Iceland (Tuscany (TSI) MAF=1.0%, CEPH Utah (CEU) MAF=0.6% (ref. 30 ); Supplementary Table 5 ). This could reflect a recent introduction of the sequence variant into the Icelandic population. STAB1 encodes stabilin-1, a transmembrane scavenger receptor expressed in a number of tissues including activated macrophages [26] . CFH At 1q31.3, in a locus containing the CFH gene, the synonymous variant rs2274700 [A] (MAF=38.62%) associates with lower LDH levels ( Table 1 ). Rs2274700 is fully correlated ( r 2 =1.00) with rs1410996 [A] (MAF=38.58%). Rs1410996 is one of a large number of sequence variants within genes of the complement system reported to associate with age-related macular degeneration [31] , [32] . In our data, the [A] allele associates with lower risk of associate with age-related macular degeneration. Mutations in CFH have also been shown to cause both atypical haemolytic uraemic syndrome [33] . CFH encodes complement factor H (FH), a key regulator of the alternative pathway of the complement system, produced and secreted in abundance by KCs [34] . FH also binds to long pentraxin 3 (PTX3) through two of FH’s SCR domains (SCR7 and SCR19-20) [35] . PTX3 influences the regulation of the complement system [36] and plays a non-redundant role in the orchestration of tissue repair and remodelling [37] . FH’s specific functions and its associations suggest that alterations of enzyme levels occur through modulation of complement activation or tissue repair and remodelling [38] . LILRB5 At 19q13.42, a locus containing LILRB5 , we observed associations of two common and modestly correlated ( r 2 =0.24) sequence variants with CK and LDH levels. The strongest signal is a missense variant rs12975366 [C] (MAF=41.62%, Asp247Gly, Asp147Gly) that associates with lower levels of both CK and LDH. A second marker, the intronic variant rs393600 [G] (MAF=25.17%) in LILRB5 , similarly associates with both CK and LDH levels. LILRB5 , encoding leukocyte immunoglobulin-like receptor subfamily B member 5, belongs to the LILR class of genes expressed on cells of myeloid lineage, and is involved in inhibition of inflammatory responses [39] , [40] . Showing association of the marker rs12975366 with CK at LILRB5 replicates previous findings [12] . HLA-DQB1 In the human leukocyte antigen (HLA) region at 6p21.3, the best association signal with LDH levels is represented by the missense variant rs17412833 [T] (MAF=13.76%, Phe119Tyr) in HLA-DQB1 . The alleles of the different HLA genes are strongly correlated to each other and often discussed as long haplotypes [41] . The HLA genes control the adaptive immune response through presentation of antigens to T cells [42] . We tested imputed HLA alleles of six of the classical HLA genes: HLA-A ; HLA-B ; HLA-C ; HLA-DQA1 ; HLA-DQB1 ; and HLA-DRB1 for association [43] . The HLA molecular type associating most strongly with serum LDH is HLA-DQB1*06:04 ( r 2 =0.53). We note that the [T] allele of rs17412833 is present in the following imputed HLA molecular types: DQB1*05:01; 05:02; 05:03; 06:04; and 06:09. HLA-DQB1 forms a part of the dimeric HLA-DQ molecule [44] . HLA-DQB1*06:04 has previously been implicated in myasthenia gravis in the Chinese [45] as well as cervical dystonia [46] . Conditional analysis shows that the HLA-DQB1*06:04 signal is fully explained by the missense variant rs17412833, but indicates that the association of rs17412833 is not explained by the HLA-DQB1*06:04 signal. NINJ1 At 9q22.31, the common intron variant rs12342201 [A] (MAF=49.45%) in NINJ1 associates with lower LDH levels ( Table 1 ). NINJ1 encodes the ninjurin-1 protein, an adhesion molecule reported to be upregulated in myeloid cells during inflammation and important in immune cell migration following neuronal injury [47] . NINJ1 expression is ubiquitous, and it has been implicated in liver function and hepatocellular senescence [48] . Muscle-linked genes associating with CK and/or LDH levels Variants at two loci are coding variants in genes that are preferentially expressed in muscle and play a role in its function. ANO5 At 11p14.3, we observed three variants in ANO5 that associate with serum CK levels. The common missense variant rs7481951 [A] (MAF=37.45%, Leu322Phe) associates with lower serum CK levels. The remaining two rare variants, the missense variant rs137854526 (MAF=0.24%, Phe578Ser), and the nonsense variant chr11:22241070:S (MAF=0.27%, Cys601X), associates with higher CK levels ( P <0.05/15 non-synonymous=3.3 × 10 −3 ). Rs137854526 occurs at a highly conserved site (GERP (ref. 27 ) =5.69). ANO5 encodes the protein anoctamin-5, a chloride channel in the endoplasmic reticulum membrane [49] , expressed mainly in skeletal and cardiac muscle. Variants in the gene, including these two rare mutations, have been reported to cause limb-girdle muscular dystrophy, which primarily affects skeletal muscle but often presents with cardiac pathologies [50] , [51] . Chr11:22241070:S shows suggestive association with heart failure (effect=1.629, P =1.0 × 10 −3 , N =11,374 cases). Two cases of compound heterozygotes for ANO5 mutations presenting with skeletal muscle dysfunction and cardiac abnormalities have been described in the literature [49] , [52] . We support this with a further two homozygotes for rare ANO5 mutations presenting with cardiovascular phenotypes. Firstly, an individual homozygous for rs137854526 and, secondly, an individual homozygous for chr11:22241070, both presenting with several cardiovascular phenotypes ( Supplementary Table 7 ). These findings provide further evidence for the effect of ANO5 variants on dysfunctions of the heart. We note another coding variant in a gene specifically expressed in muscle has a P value just above the significance threshold. The common missense variant in CACNG1 rs1799938 [A] (MAF=10.64%, Gly196Ser) suggestively associates with CK levels ( P =3.2 × 10 −7 ; effect=0.046). CACNG1 encodes the γ subunit of a 1,4-dihydropyridine (DHPR) -sensitive calcium channel, preferentially expressed in skeletal muscle [53] . Other signals associating with CK and/or LDH Levels The three remaining association signals are at loci without any obvious causative gene. We observed a signal at 11p11.2 associating with lower serum LDH levels, represented by a large group of 276 correlated markers ( r 2 >0.6; Supplementary Data 1 ). The marker showing the strongest association is the common intergenic variant rs2930191 [A] (MAF=37.22%). At 12q24.13, the low-frequency variant chr12:110830276:S (MAF=2.09%) associates significantly with lower LDH levels, and suggestively with CK levels. Finally, at 13q22.1, the common variant rs7318906 [A] (MAF=47.08%) associates with decreased CK levels. We used GTEx Portal’s eQTL Browser to assess whether any of our reported variants affected gene expression. None of the 25 markers we discussed in the current study was directly reported or correlated ( r 2 >0.2) to any GTEX cis-eqtl ( P <1 × 10 –5 ). Signals observed specifically in statin takers We examined statin usage, stratifying our CK and LDH measurements by statin intake. Prescription data for statins were available for a period of time ranging from 2003 to 2009 and the stratified analysis therefore only included blood measurements from this interval. No additional signals were detected ( Supplementary Figs 1–4 ). Our data showed no indication of the overall results being driven by individuals treated by statins, or any genetic susceptibility to statin side effects, for any of the loci in question ( Supplementary Tables 8 and 9 ). Furthermore, the reported variant rs4363657 in SLCO1B1 showed no effect on any of the tested phenotypes ( Supplementary Table 10 ). Advantages of whole-genome sequencing For the 25 reported variants, twenty were present in the 1000G data set ( Supplementary Table 11 ). Of these, three could not be imputed, and a further three showed very low correlation ( r 2 <0.64) between the directly typed and the 1000G imputed phenotypes. Fourteen variants showed high correlation between directly typed and imputed genotypes ( r 2 ⩾ 0.8) and could therefore plausibly have been discovered using only 1000G imputation. Five variants were not present in 1000G, but had correlates ( r 2 >0.6) within the data set ( Supplementary Table 12 ). Of these, four showed good correlation ( r 2 >0.6) between imputed and correlated genotypes, and could, therefore, have shown association with CK or LDH levels in a study relying purely on a 1000G imputation data set. We therefore report seven variants that could not have been discovered using a 1000G imputation set. Elevation of serum enzyme levels can be a result of two separate processes; increased leakage from tissue into the serum, or reduced clearance [54] . Furthermore, observations of altered serum enzyme levels can result from a change in enzymatic activity. We report variants affecting serum enzyme levels through all three mechanisms. Our discovery of a high number of genes linked to immune response is consistent with the MPS’s role in clearing debris and foreign material from the bloodstream, including through receptor-mediated endocytosis of short-lived cellular enzymes [55] , [56] . Although the MPS has been implicated, the specific receptors responsible for uptake of serum enzymes have not yet been identified [24] . Nonspecific receptors, responsible for uptake of several enzymes, have been postulated [24] , [57] . We report a number of variants in genes expressed preferentially in phagocytic cells, notably hepatic KCs, which affect levels of serum enzymes. The protein products encoded by CD163 and STAB1 , and LILRB5 are all scavenger receptors expressed by macrophages [58] , [59] , and could be the unidentified receptors responsible for endocytosis of serum enzymes by cells of the MPS. Non-synonymous variants in ANO5 associates with serum CK levels, consistent with the fact that serum CK levels are largely influenced by leakage of CK from damaged myocytes [60] . The results of this study underscore the diversity in sources of variation of serum enzyme levels, each of which are influenced by sequence variants, and must be kept in mind when interpreting the measurements. Population Measurements of serum CK levels were available for a total of 63,159 Icelanders. Of these, 35,623 were genotyped using Illumina chips and imputed using long-range-phased haplotypes. Genotype probabilities were calculated for 27,536 individuals based on genetic information available for first and second-degree relatives. Measurements of serum LDH levels were available for a total of 98,585 individuals, 52,581 of whom were chip-typed using Illumina chips, and 46,004 of whom had genotype probabilities calculated. All individuals had provided consent, and the study was approved by the Data Protection Commission of Iceland and the Icelandic National Bioethics Committee. Stratification by statin intake CK and LDH measurements were stratified by statin intake. CK measurements were available for 8,900 statin takers (CK on statin =5,207; CK off statin =6,877), and LDH measurements were available for 9,851 statin takers (LDH on statin =6,266; LDH off statin =6,877), respectively, with an overlap of 7,534 individuals. These cohorts were used to test sequence variants for association with serum enzyme levels during and outside of times of statin use. Serum enzyme measurements Serum enzyme measurements were obtained from three laboratories in Iceland: The Laboratory of the Icelandic National University Hospital; The Icelandic Medical Center Laboratory in Mjodd; and Akureyri Hospital. We used measurements of serum CK ( N =63,159, geometric mean=211.1), and LDH ( N =98,585, geometric mean=113.1). Additional measurement characteristics can be found in Supplementary Table 13 . Serum levels were adjusted for sex, age and laboratory of origin. When multiple measurements were available for an individual, the mean adjusted value was used. Whole-genome sequencing and Illumina single-nucleotide polymorphism chip genotyping The process used to whole-genome sequence the 2,636 Icelanders, and the subsequent imputation from which the data for this analysis were generated has been extensively described in a recent publication [14] . Association analysis All serum enzyme measurements were corrected for age, sexand laboratory of origin, and were subsequently standardized to have a normal distribution. To test for association between quantitative traits and sequence variants, a generalized form of linear regression was used (see Supplementary Note 1 ). The quantitative trait was used as the response variable and the expected allele count (gene dosage) as the covariate. In the regression analysis of CK/LDH, we used genealogy information and assume a variance covariance matrix proportional to the kinship matrix (see Supplementary Note 1 ). To account for relatedness and stratification within the case and control sample sets, we applied the method of genomic control [61] . The inflation factor λ g of the χ 2 statistics was estimated on the basis of a set of about 300,000 common variants distributed across the genome, and P values were adjusted by dividing the corresponding χ 2 values by this factor. The genomic control was calculated to be λ =1.16 for CK and 1.22 for LDH ( Supplementary Figs 34 and 35 ). Significance thresholds Sequence variants were weighted according to their prior probability of affecting gene function. Thresholds for genome-wide significance were applied, depending on variant class, as described by Sveinbjornsson et al . [18] . The type I error rate of 0.05 was allocated equally between three classes of variants; loss-of-function ( N =6,476), missense ( N =100,502) and other variants ( N =23,854,999). This yielded class-specific Bonferroni genome-wide significance thresholds of 2.6 × 10 −6 , 1.7 × 10 −7 and 7.0 × 10 −10 , respectively. Sanger sequencing and reimputation Two sequence variants were poorly imputed due to a low number of sequenced carriers in the original Icelandic data set. A group of suspected carriers and non-carriers of the missese variants rs145987658 in CKM (info=0.63) and rs150956780 in STAB1 (info=0.58) were Sanger sequenced, and reimputation was subsequently carried out. Imputation information following reimputation increased for both variants. Fraction of variance explained Fractions of CK and LDH variance explained by the reported variants were calculated using the formula 2 f (1− f ) a 2 , where f =MAF and a =effect. Accession codes: European Variant Archive: PRJEB8636. How to cite this article: Kristjansson, R. P. et al . Common and rare variants associating with serum levels of creatine kinase and lactate dehydrogenase. Nat. Commun. 7:10572 doi: 10.1038/ncomms10572 (2016).